The SH2 domain of Abl kinases regulates kinase autophosphorylation by controlling activation loop accessibility The activity of protein kinases is regulated by multiple molecular mechanisms, and their disruption is a common driver of oncogenesis. A central and almost universal control element of protein kinase activity is the activation loop that utilizes both conformation and phosphorylation status to determine substrate access. In this study, we use recombinant Abl tyrosine kinases and conformation-specific kinase inhibitors to quantitatively analyse structural changes that occur after Abl activation. Allosteric SH2–kinase domain interactions were previously shown to be essential for the leukemogenesis caused by the Bcr–Abl oncoprotein. We find that these allosteric interactions switch the Abl activation loop from a closed to a fully open conformation. This enables the trans -autophosphorylation of the activation loop and requires prior phosphorylation of the SH2–kinase linker. Disruption of the SH2–kinase interaction abolishes activation loop phosphorylation. Our analysis provides a molecular mechanism for the SH2 domain-dependent activation of Abl that may also regulate other tyrosine kinases. The activation state of protein kinases is controlled by a number of molecular mechanisms [1] , [2] . The deregulation of these mechanisms by point mutations, translocations, deletions or duplications often results in the overactivation of kinases, which can lead to cancer and other malignancies [3] . Within the family of human cytoplasmic tyrosine kinases with its 34 members, inhibition and activation is regulated through various dynamic intramolecular protein–protein interactions between the SH3, SH2 and kinase domains (KDs) [1] , [4] , [5] . Abelson tyrosine kinase (Abl, encoded by the human ABL1 gene) is ubiquitously expressed and involved in several cellular processes [6] . Abl kinase activity is autoinhibited through various intramolecular interactions involving its SH3 and SH2 domains, as well as its amino-terminal myristoyl group [7] , [8] , [9] . Loss of autoinhibition occurs by fusion with the breakpoint cluster region (Bcr) protein that results from the Philadelphia chromosome translocation. This leads to the formation of Bcr–Abl fusion protein, the main driver of chronic myeloid leukaemia [10] and target of the first and largest class of kinase inhibitors currently in clinical use [11] , [12] . Studies on activated Abl and Fes kinases showed that active cytoplasmic tyrosine kinases are not fully disassembled, but that distinct domain–domain interactions are newly formed on activation to sustain in vitro and cellular activities [13] , [14] . In both kinases, a large intramolecular interface of the small subdomain (N-lobe) of the KD with its SH2 domain was observed [14] , [15] , [16] . The physiological significance of this interface of Bcr–Abl was highlighted by the dramatic reduction in transformation and loss of leukemogenesis on disruption of the SH2–kinase interaction by a single point mutation in the SH2 domain (I164E) in a chronic myeloid leukaemia mouse model [17] . Targeting of the SH2–KD interface with an engineered high-affinity monobody inhibited Bcr–Abl kinase activity and transformation [17] ; thus, this site was validated as an allosteric drug target [18] . The molecular mechanism for kinase activation by binding of the SH2 domain to the KD is not understood because high-resolution structures of active Abl have not been determined. Another characteristic, but poorly understood, property of active Abl is its high level of tyrosine phosphorylation, whereas autoinhibited Abl is not phosphorylated on tyrosine residues [5] , [19] , [20] . Few phosphorylation sites have been studied in more detail, including Tyr-412 and Tyr-245. Tyr-412 is located in the activation loop of the KD. The activation loop is a flexible loop that can adopt different conformations and regulate access of the substrate to the catalytic cleft [1] , [21] . An open conformation of the activation loop enables substrate binding and is often stabilized by the phosphorylation of one or several residues. However, certain kinases lack activation loop phosphorylation sites, such as CaMKII, or the phosphorylation, for example, in c-Kit or EGFR (epidermal growth factor receptor), can be dispensed for full kinase activation [22] . On Abl activation, the activation loop gets phosphorylated at Tyr-412 (refs 23 , 24 ). A structural analysis showed that phosphorylation stabilizes the open conformation of Abl [25] . Despite these results, the isolated Abl KD does not require phosphorylation for in vitro kinase activity [26] . A second phosphorylation site, Tyr-245, is located in the SH2–kinase linker, and its phosphorylation impairs the autoinhibitory binding of the SH3 domain to the SH2–KD linker [8] . Mutation of Tyr-245 impairs Abl activation [23] . However, it remains unclear whether Tyr-412 and Tyr-245 phosphorylations are mere stabilizers of the active conformation and how SH2 domain-mediated allosteric activation affects these phosphorylation sites. We show that structural and cellular properties of active Abl can be recapitulated with bacterially expressed highly purified Abl proteins. By using type-1 and type-2 Abl kinase inhibitors as a reference, we show that the formation of the SH2–KD interface is a critical switch to fully open and expose the Abl activation loop for efficient autophosphorylation. Bacterially expressed Abl SH2–KD unit proteins Many studies that led to key insights into Abl regulation used proteins that were expressed in mammalian cell lines; furthermore, these proteins had limited purity, were difficult to quantify and contained heterogeneous post-translational modifications [7] , [9] , [17] , [23] , [24] . To overcome these shortcomings, we adapted an efficient Escherichia coli expression system for Abl and related kinases [27] . The SH2–KD unit and KD alone of human Abl were purified to homogeneity by affinity and ion-exchange chromatography with excellent final yields of 3–15 mg per liter of culture ( Fig. 1a–c ). We also purified SH2–KD proteins carrying mutations in the SH2 domain. These mutations were predicted to decrease the interaction with the KD N-lobe (I164E; refs 14 , 17 ), increase this interaction (T231R; ref. 28 ) or show impaired phosphotyrosine binding (S173N; ref. 17 ; Fig. 1b,c ). In addition, kinase-defective (D382N; ref. 8 ) proteins and two phosphorylation site mutants Y412F (refs 23 , 24 ) and Y245F (refs 23 ) were purified ( Fig. 1c ). All purified proteins were monomeric in gel filtration analysis and monodispersed in multi-angle light-scattering analysis ( Fig. 1d ; Supplementary Fig. 1 ). The far-ultraviolet circular dichroism spectra of SH2–KD wt (wild type) and I164E were virtually identical, indicating that disrupting the SH2-kinase interface had no major impact on protein folding or stability ( Supplementary Fig. 2 ). Mass spectrometric analysis was in close agreement with the expected mass of the unmodified proteins and showed no evidence of tyrosine phosphorylation ( Supplementary Fig. 3 ). All data indicate that the bacterially expressed SH2–KD proteins are unphosphorylated and have excellent properties for quantitative enzymatic and biophysical studies. 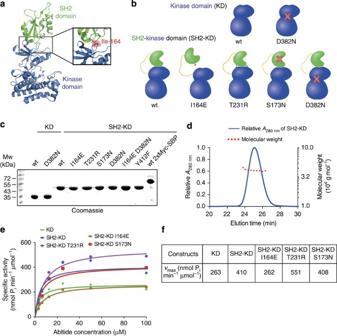Figure 1: Biophysical and enzymatic analysis of purified bacterially expressed Abl mutants. (a) The structure of the active SH2–KD unit of human Abl (Protein Data Bank (PDB) entry 1OPL, molecule B). Ile-164 is a central residue in the SH2–KD interface and is shown in red. (b) Schematic representation of the central mutants used in this study. Red crosses indicate inactivating mutations in either the KD (D382N mutation in the catalytic loop) or SH2 domain (S173N mutation in the FLVRES motif). The T231R mutation was predicted to form a salt bridge with Glu-294 in the KD and stabilize the SH2–kinase interface. (c) Coomassie staining of 20 μg of bacterially expressed and purified Abl mutants used for this study. (d) Gel filtration coupled with a multi-angle light-scattering analysis of SH2–KD wt. The analysis of SH2–KD mutants is shown inSupplementary Fig. 1. The absorption at 280 nm (blue solid line, leftyaxis) and molecular weight (red dotted line, rightyaxis) are shown. (e) Purified Abl mutant proteins were assayed for kinase activity by measuring incorporation of32P into an optimal Abl substrate peptide (Abltide). Averages of a representative experiment with two technical replicates are shown. The experiment was repeated twice. (f)vmaxwas calculated after fitting the kinase activity data to the Michaelis–Menten equation. Additional enzymatic parameters are shown inSupplementary Table 1. Figure 1: Biophysical and enzymatic analysis of purified bacterially expressed Abl mutants. ( a ) The structure of the active SH2–KD unit of human Abl (Protein Data Bank (PDB) entry 1OPL, molecule B). Ile-164 is a central residue in the SH2–KD interface and is shown in red. ( b ) Schematic representation of the central mutants used in this study. Red crosses indicate inactivating mutations in either the KD (D382N mutation in the catalytic loop) or SH2 domain (S173N mutation in the FLVRES motif). The T231R mutation was predicted to form a salt bridge with Glu-294 in the KD and stabilize the SH2–kinase interface. ( c ) Coomassie staining of 20 μg of bacterially expressed and purified Abl mutants used for this study. ( d ) Gel filtration coupled with a multi-angle light-scattering analysis of SH2–KD wt. The analysis of SH2–KD mutants is shown in Supplementary Fig. 1 . The absorption at 280 nm (blue solid line, left y axis) and molecular weight (red dotted line, right y axis) are shown. ( e ) Purified Abl mutant proteins were assayed for kinase activity by measuring incorporation of 32 P into an optimal Abl substrate peptide (Abltide). Averages of a representative experiment with two technical replicates are shown. The experiment was repeated twice. ( f ) v max was calculated after fitting the kinase activity data to the Michaelis–Menten equation. Additional enzymatic parameters are shown in Supplementary Table 1 . Full size image Recombinant SH2–KD recapitulates regulation by SH2 domain We performed in vitro enzyme-kinetic experiments using an optimal Abl substrate peptide ( Fig. 1e ). We observed an increase in the v max of SH2–KD when compared with KD. As expected, the I164E mutation nullified this increase, whereas v max was further increased by the T231R mutation ( Fig. 1f ). The S173N mutation that renders the SH2 domain incapable of binding to phosphotyrosine ligands had the same v max as SH2–KD wt ( Fig. 1f ). The Michaelis–Menten constant ( K M ) was similar for all tested mutants ( Supplementary Table 1 ). Importantly, the observed K M values and relative increases/decreases in v max with the SH2 mutations are in close agreement with the data of immune-complex kinase assays that used full-length Bcr–Abl, full-length Abl or SH2–KD proteins that were transiently expressed in mammalian cell lines [14] , [17] , [28] . Despite the lack of tyrosine phosphorylation, the bacterially expressed Abl proteins exhibited robust in vitro kinase activity, in line with the results for Abl KDs purified from insect cells [26] . These results showed that previous observations on the allosteric role of the SH2 domain in cells could be recapitulated in vitro with bacterially expressed Abl proteins; thus, our subsequent experimental procedures were validated. SH2–KD mutant structures by small-angle X-ray scattering It is important to determine whether the utilized SH2–KD proteins maintain their conformation when the SH2 domain is bound to the KD N-lobe in the absence of other domains. We used small-angle X-ray scattering (SAXS) to analyse the conformations of KD, SH2–KD wt and their mutants in solution. The SAXS data revealed increasingly extended conformations in KD (maximum size D max =~70 Å) to SH2–KD wt ( D max =~95 Å) to SH2–KD I164E ( D max =~110 Å; Fig. 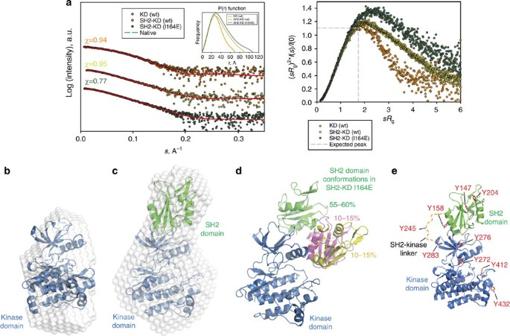Figure 2: Structural analysis of SH2–KD unit and mapping of phosphorylation sites. (a) Experimental (dots) and calculated (red lines) SAXS data for KD, SH2–KD wt and SH2–KD I164E, respectively.P(r) functions (insert, left panel) and normalized Kratky plots (right panel) are shown. The expected peak (grey dashed line) represents the theoretical peak assuming an ideal Guinier region of a globular particle. (b,c) Theab initioshape reconstructions of KD (b) and SH2–KD wt (c) were superimposed on their crystal structures (PDB entries, 1OPJ for KD and 1OPL molecule B for SH2–KD wt). The normalized spatial discrepancy (NSD) values (computed using SUPCOMB47) were 0.9351 and 0.9294 for KD and SH2–KD, respectively. NSD values lower than 1 are indicative of a well-fit superimposition. (d) Flexible characterization of SH2–KD (I164E) showing an ensemble of three possible positions for the SH2 domain based on EOM analysis. (e) The positions of phosphorylation sites mapped by mass spectrometry after SH2–KD wt autophosphorylation are shown as red sticks on the structure of SH2–KD (PDB entry 1OPL, molecule B). The SH2–kinase linker is shown as an orange dotted line. Details on phosphorylation sites are given inTable 1. 2a , left panel; Supplementary Table 2 ). The low-resolution ab initio shape reconstructions for KD and SH2–KD wt superimposed well with the available crystal structures [8] , [13] , [26] ( Fig. 2b,c ). These results indicated that the SH2 domain is bound to the N-lobe of the KD in SH2–KD. These data are also in agreement with previous SAXS analyses of an activated, but catalytically inactive, SH3-SH2–KD construct [13] . For the SH2–KD mutant I164E, the data suggested significant domain rearrangements, and rigid body modelling using the available domain structures did not provide a satisfactory fit ( Supplementary Fig. 4 ). Thus, the potential flexibility of the mutant and the scattering data was analysed in terms of co-existing conformer ensembles, which provided an improved fit with the data ( Fig. 2a ). Furthermore, the Kratky plot ( Fig. 2a , right panel) suggested an increase in the flexibility in the I164E mutant because a shift from the expected peak was observed. The selected ensembles that elucidated the conformational space of possible SH2 domain positions with respect to the KD are displayed in Fig. 2d . The analysis also indicated that the I164E mutant may partially dimerize in solution because the selected ensembles contained a small percentage (10–15%) of dimers ( Supplementary Fig. 5 ). In contrast, the T231R mutant protein, addition of type-1 or type-2 tyrosine kinase inhibitors (dasatinib or nilotinib, respectively) or the phosphorylation of SH2–KD, did not produce significant differences in the SH2–KD wt (data not shown). Collectively, the SAXS analysis indicated that the SH2 is stably bound to the N-lobe of the KD and only mutational disruption of the interface results in conformational changes. Therefore, the bacterially expressed proteins used in this study structurally recapitulate the active Abl conformation observed with larger constructs in previous studies. Figure 2: Structural analysis of SH2–KD unit and mapping of phosphorylation sites. ( a ) Experimental (dots) and calculated (red lines) SAXS data for KD, SH2–KD wt and SH2–KD I164E, respectively. P ( r ) functions (insert, left panel) and normalized Kratky plots (right panel) are shown. The expected peak (grey dashed line) represents the theoretical peak assuming an ideal Guinier region of a globular particle. ( b , c ) The ab initio shape reconstructions of KD ( b ) and SH2–KD wt ( c ) were superimposed on their crystal structures (PDB entries, 1OPJ for KD and 1OPL molecule B for SH2–KD wt). The normalized spatial discrepancy (NSD) values (computed using SUPCOMB [47] ) were 0.9351 and 0.9294 for KD and SH2–KD, respectively. NSD values lower than 1 are indicative of a well-fit superimposition. ( d ) Flexible characterization of SH2–KD (I164E) showing an ensemble of three possible positions for the SH2 domain based on EOM analysis. ( e ) The positions of phosphorylation sites mapped by mass spectrometry after SH2–KD wt autophosphorylation are shown as red sticks on the structure of SH2–KD (PDB entry 1OPL, molecule B). The SH2–kinase linker is shown as an orange dotted line. Details on phosphorylation sites are given in Table 1 . Full size image Mapping of SH2–KD autophosphorylation sites Active Abl is phosphorylated on several sites in cells; therefore, we mapped SH2–KD autophosphorylation sites in vitro by mass spectrometry after incubating the protein with excess ATP. Among the 24 tyrosines that are present in the SH2–KD protein, we found that nine tyrosines became phosphorylated ( Fig. 2e ; Table 1 ). All identified phosphorylation sites were found highly annotated in the PhosphoSite repository ( http://www.phosphosite.org/ ) and were previously identified in multiple phospho-proteomics data sets from Bcr–Abl-expressing cells or other cancer cell lines ( Table 1 ). Very few additional Abl tyrosine phosphorylation sites were reported on PhosphoSite, and all of these sites had a low record count. These results showed that Abl retained its specificity in vitro because all of the in vitro phosphorylation sites were also reported in cells. This analysis validates previous functional data that concentrated on the highly phosphorylated Tyr-412 and Tyr-245 sites. Table 1 Identified in vitro autophosphorylation sites of the Abl SH2–KD wt protein. Full size table SH2 domain is required for activation loop autophosphorylation First, we analysed the activation mechanism using unphosphorylated kinases. We incubated KD and SH2–KD proteins with ATP and monitored the increase in total tyrosine phosphorylation over time using a quantitative dot-blot assay system. Surprisingly, KD was completely defective in autophosphorylation ( Fig. 3a–c ; Supplementary Fig. 6 ), despite robust kinase activity towards an exogenous peptide substrate ( Fig. 1e ). Extended incubation times of up to 3 h did not lead to a significant increase in kinase autophosphorylation (data not shown). In stark contrast, SH2–KD showed a fast and robust increase in autophosphorylation that was further increased with the T231R mutation. However, the I164E mutation showed a strong decrease in autophosphorylation kinetics ( Fig. 3a–c ; Supplementary Fig. 6 ). The S173N mutant protein showed no differences when compared with the wild-type protein, indicating that total Abl kinase autophosphorylation does not require phosphotyrosine binding of the SH2 domain ( Fig. 3a ; Supplementary Fig. 6 ). 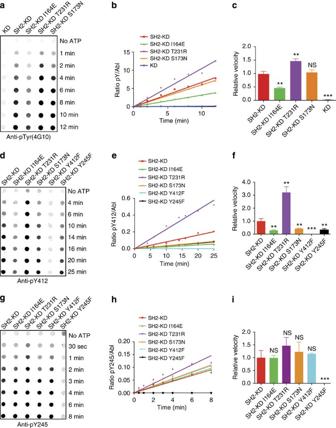Figure 3: Disruption of the SH2–kinase interface impairs Abl autophosphorylation. (a,d,g) The indicated Abl proteins were incubated for the indicated times with ATP, dot blotted and incubated with antibodies for total pY (a), pY412 (d) and pY245 (g). The phosphotyrosine antibodies co-incubated with anti-Abl or anti-5xHis antibodies (Supplementary Fig. 6) were used to normalize the data for possible unequal loading or transfer of recombinant protein samples. (b,e,h) Normalized total pY, pY412 and pY245 signals were plotted over incubation time of the autophosphorylation reactions, and the slopes (relative velocities) of linear fits were calculated. (c,f,i) The relative velocities of autophosphorylation reactions of the indicated SH2–KD mutants from three independent experiments (biological repeats) are shown. Averages±s.d. are plotted. For each data set, the SH2–KD wt was set to 1.0. Significance levels in comparison with the SH2–KD wt are indicated (NS, not significant; **P<0.01, ***P<0.001, unpairedt-test). Figure 3: Disruption of the SH2–kinase interface impairs Abl autophosphorylation. ( a , d , g ) The indicated Abl proteins were incubated for the indicated times with ATP, dot blotted and incubated with antibodies for total pY ( a ), pY412 ( d ) and pY245 ( g ). The phosphotyrosine antibodies co-incubated with anti-Abl or anti-5xHis antibodies ( Supplementary Fig. 6 ) were used to normalize the data for possible unequal loading or transfer of recombinant protein samples. ( b , e , h ) Normalized total pY, pY412 and pY245 signals were plotted over incubation time of the autophosphorylation reactions, and the slopes (relative velocities) of linear fits were calculated. ( c , f , i ) The relative velocities of autophosphorylation reactions of the indicated SH2–KD mutants from three independent experiments (biological repeats) are shown. Averages±s.d. are plotted. For each data set, the SH2–KD wt was set to 1.0. Significance levels in comparison with the SH2–KD wt are indicated (NS, not significant; ** P <0.01, *** P <0.001, unpaired t -test). Full size image Next, we analysed autophosphorylation kinetics using phosphorylation site-specific antibodies. We chose to follow the phosphorylation of Tyr-412 in the activation loop and Tyr-245 in the SH2–kinase linker because both sites are important for Abl activation [23] , [24] and reliable phosphorylation site-specific antibodies were available. Autophosphorylation of Tyr-412 was strongly decreased in the I164E mutant protein and almost nullified with a second mutation of the SH2–kinase interface (S162K) when compared with SH2–KD wt; however, the T231R mutant protein showed a strong increase in phosphorylation kinetics at Tyr-412, paralleling the findings on total tyrosine phosphorylation ( Fig. 3d–f ; Supplementary Figs 6 and 7 ). In contrast, disrupting or enhancing SH2–kinase interactions did not affect the phosphorylation at Tyr-245 ( Fig. 3g–i ; Supplementary Fig. 6 ). Notably, Tyr-245 phosphorylation seemed to precede Tyr-412 phosphorylation because the process began earlier and showed a steeper incline ( Fig. 3d–g ; Supplementary Fig. 8 ). Thus, we tested the possible interdependence of these two phosphorylation events using Y412F and Y245F mutant proteins. Apart from excluding crossreactivity of the two phospho-specific antibodies, the Y245F protein reduced the autophosphorylation kinetics at Tyr-412 but did not show reduced activity for an exogenous peptide substrate ( Fig. 3d–f ; Supplementary Fig. 9 ). However, the ability of the Y412F protein to autophosphorylate Tyr-245 was unchanged ( Fig. 3g–i ). Prior Tyr-245 phosphorylation could enhance Tyr-412 phosphorylation by the binding of phosphotyrosine-245 to the SH2 domain; therefore, we also tested the effect of the S173N mutation that renders the SH2 domain incapable of phosphotyrosine binding. As expected, the S173N mutant protein autophosphorylated Tyr-245 with the same kinetic as the wild-type protein ( Fig. 3g–i ). In contrast, Tyr-412 phosphorylation was strongly impaired by the S173N mutation ( Fig. 3d–f ). In summary, these experiments show that the SH2–KD interface is a major determinant that enables Abl autophosphorylation. The Abl KD is defective in the autophosphorylation of the activation loop in the absence of SH2–kinase interaction. It is important to note that these effects are markedly more pronounced than the differences in v max for phosphorylation of a peptide substrate ( Fig. 1e ). In addition, the autophosphorylation experiments were completed with enzyme concentrations that are well below the K M for substrate peptides (see Supplementary Table 1 ). Therefore, the dramatic differences in activation loop autophosphorylation are unlikely to be caused by differences in the in vitro kinase activity of the mutant proteins. Efficient trans -autophosphorylation requires the SH2 domain Abl autophosphorylation can occur intramolecularly (in ‘ cis ’) or intermolecularly (in ‘ trans ’). We found that the specific activity of autophosphorylation of the SH2–KD wt and I164E proteins increased linearly with kinase concentrations ( Supplementary Fig. 10 ). This observation supports an expected first-order reaction for autophosphorylation in the trans but not cis autophosphorylation process. We speculated that one or several phosphorylation sites in the KD might be sterically less accessible because the KD protein did not show a strong impairment of in vitro kinase activity, despite its inability to autophosphorylate. To test this hypothesis, we co-incubated pairs of active (wt) and catalytically deficient (D382N) KD and SH2–KD proteins and then monitored the trans -phosphorylation of the D382N (substrate) protein by the wt (kinase) protein on Tyr-412 by quantitative immunoblotting ( Fig. 4a ). Incubation of active KD wt with inactive SH2–KD D382N showed robust trans -phosphorylation of the SH2–KD D382N activation loop, whereas SH2–KD D382N alone did not show autophosphorylation ( Fig. 4b ; Supplementary Fig. 11 ). In contrast, incubation of SH2–KD wt with KD D382N did not lead to a significant increase in Tyr-412 phosphorylation above background levels ( Fig. 4a,b ). Using the same experimental design, we showed that the robust phosphorylation on Tyr-412 of SH2–KD D382N by KD wt was abolished by the disruption of the SH2–KD interface by the I164E mutation ( Fig. 4c–f ). Both experiments showed that the SH2–KD interface has a major impact on the accessibility of Tyr-412 in the activation loop because the absence of the SH2 domain or mutational disruption of the SH2–kinase interface renders the activation loop a poor substrate for trans -phosphorylation. 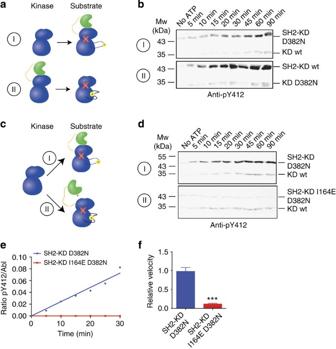Figure 4: The activation loop is a poor substrate fortrans-autophosphorylation in the absence of the SH2–kinase interface. (a,c) Models illustrating the two combinations of mutants tested inb,dare shown. (b,d) The indicated KD and SH2–KD proteins were co-incubated for the indicated times and analysed by immunoblotting with an anti-pY412 antibody and anti-5xHis antibody (Supplementary Fig. 6). All samples were loaded on the same membrane to allow for direct comparisons. The data are shown as two panels for graphical convenience only. (e) Normalized pY412 signals were plotted over incubation time of the autophosphorylation reactions, and the slopes (relative velocities) of linear fits were calculated. (f) The relative velocities for the autophosphorylation reactions of the indicated SH2–KD mutants from three independent experiments (biological repeats) are shown. Averages±s.d. are plotted. The SH2–KD wt was set to 1.0. Significance levels in comparison with the SH2–KD wt are indicated (***P<0.001, unpairedt-test). Uncropped blots are shown inSupplementary Fig. 13. Figure 4: The activation loop is a poor substrate for trans -autophosphorylation in the absence of the SH2–kinase interface. ( a , c ) Models illustrating the two combinations of mutants tested in b , d are shown. ( b , d ) The indicated KD and SH2–KD proteins were co-incubated for the indicated times and analysed by immunoblotting with an anti-pY412 antibody and anti-5xHis antibody ( Supplementary Fig. 6 ). All samples were loaded on the same membrane to allow for direct comparisons. The data are shown as two panels for graphical convenience only. ( e ) Normalized pY412 signals were plotted over incubation time of the autophosphorylation reactions, and the slopes (relative velocities) of linear fits were calculated. ( f ) The relative velocities for the autophosphorylation reactions of the indicated SH2–KD mutants from three independent experiments (biological repeats) are shown. Averages±s.d. are plotted. The SH2–KD wt was set to 1.0. Significance levels in comparison with the SH2–KD wt are indicated (*** P <0.001, unpaired t -test). Uncropped blots are shown in Supplementary Fig. 13 . Full size image Activation loop-active conformation induced by SH2 domain To quantitatively assess the conformation of the activation loop in Abl KD and SH2–KD, we used kinase inhibitors to induce either an open or closed conformation of the activation loop. Analysis of the Abl KD crystal structures in complex with imatinib (a type-2 inhibitor) showed the activation loop to be in an inward-facing closed conformation, and Tyr-412 acted as a pseudo-substrate and was not accessible for phosphorylation [26] , [29] . However, crystal structures of dasatinib (a type-1 inhibitor) with the KD of Abl and several other kinases showed that the activation loop was in an extended and open conformation with Tyr-412 being exposed to solvent [30] . Both imatinib- and dasatinib-induced activation loop conformations were confirmed using solution nuclear magnetic resonance techniques [31] . We prepared both KD and SH2–KD proteins in complex with imatinib and dasatinib that were unable to autophosphorylate and were catalytically inactive ( Supplementary Fig. 11 ). We used these kinase–drug complexes as trans -phosphorylation substrates along with (catalytically deficient) KD D382N or SH2–KD D382N and monitored the phosphorylation of Tyr-412 over time ( Fig. 5a–f ; Supplementary Fig. 12 ). Similar to the KD–imatinib complex, KD D382N was defective in Tyr-412 phosphorylation, whereas KD–dasatinib was phosphorylated readily at Tyr-412 ( Fig. 5a–c ; Supplementary Fig. 12 ). This result indicates that the activation loop in KD is in a closed conformation similar to the imatinib complex. The same donor kinase was used to monitor the phosphorylation of SH2–KD. We included a 2xMyc-SBP tag in the (active) SH2–KD wt constructs that allowed us to distinguish the two co-incubated proteins using their different molecular weights ( Fig. 5d ). In contrast to the results obtained with KD D382N, SH2–KD D382N showed phosphorylation at Tyr-412 to a similar degree as the SH2–KD–dasatinib complex, whereas the SH2–KD–imatinib complex was strongly impaired in trans -phosphorylation at Tyr-412 ( Fig. 5d–f ; Supplementary Fig. 12 ). This result indicates that the activation loop in SH2–KD is similar to the dasatinib complex and exists in a fully open conformation that is accessible. The robust, albeit not complete, rescue of trans -phosphorylation of the KD–dasatinib complex when compared with SH2–KD D382N also indicates that there is no principal requirement for the SH2 domain to enable trans -autophosphorylation. This mechanism would be expected if the SH2 domain was involved in kinase dimerization. 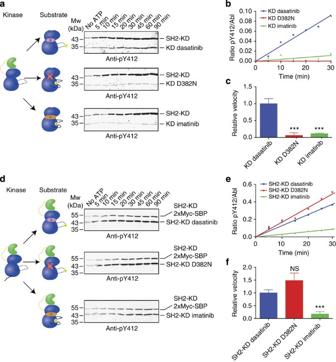Figure 5: The SH2 domain induces a fully active conformation of the activation loop. (a,d) Active SH2–KD was incubated with dasatinib-, catalytically inactive- or imatinib-bound KD (a) and SH2–KD (d) proteins for the indicated times and then analysed by immunoblotting with an anti-pY412 antibody and anti-5xHis antibody (Supplementary Fig. 6). All samples were loaded on the same membrane to allow for direct comparisons. The data are shown as three panels for graphical convenience only. (b,e) The normalized pY412 signals of immunoblots ina,dwere plotted over incubation time for thetrans-phosphorylated substrate (lower band) of the reactions, and the slopes (relative velocities) of linear fits were calculated. (c,f) The relative velocities oftrans-phosphorylation reactions from three independent experiments (biological repeats) are shown. Averages±s.d. are plotted. For each data set, the dasatinib complex was set to 1.0. Significance levels in comparison with the dasatinib-bound KD (c) or SH2–KD (f) are indicated (NS, not significant; ***P<0.001, unpairedt-test). Uncropped blots are shown inSupplementary Fig. 13. Figure 5: The SH2 domain induces a fully active conformation of the activation loop. ( a , d ) Active SH2–KD was incubated with dasatinib-, catalytically inactive- or imatinib-bound KD ( a ) and SH2–KD ( d ) proteins for the indicated times and then analysed by immunoblotting with an anti-pY412 antibody and anti-5xHis antibody ( Supplementary Fig. 6 ). All samples were loaded on the same membrane to allow for direct comparisons. The data are shown as three panels for graphical convenience only. ( b , e ) The normalized pY412 signals of immunoblots in a , d were plotted over incubation time for the trans -phosphorylated substrate (lower band) of the reactions, and the slopes (relative velocities) of linear fits were calculated. ( c , f ) The relative velocities of trans -phosphorylation reactions from three independent experiments (biological repeats) are shown. Averages±s.d. are plotted. For each data set, the dasatinib complex was set to 1.0. Significance levels in comparison with the dasatinib-bound KD ( c ) or SH2–KD ( f ) are indicated (NS, not significant; *** P <0.001, unpaired t -test). Uncropped blots are shown in Supplementary Fig. 13 . Full size image Collectively, these results show that the SH2 domain acts to allosterically activate Abl by converting the KD from an intrinsically inactive conformation to an active conformation in which the activation loop is fully exposed for subsequent phosphorylation to stabilize the active kinase conformation ( Fig. 6 ). 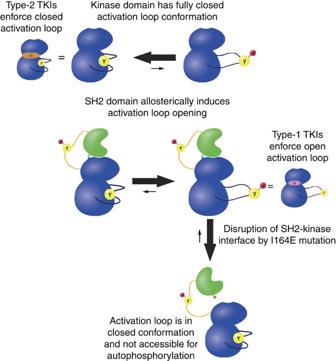Figure 6: The experimental observations of this study are summarized in a graphical model. The Abl KD has a predominantly inactive activation loop conformation that is similar to the conformation once imatinib or other type-2 kinase inhibitors are bound (upper panel). On formation of the SH2–kinase interface, the equilibrium is shifted to a predominantly open activation loop similar to the conformation once dasatinib or other type-1 inhibitors bind to the KD (lower panel). Disruption of the SH2–kinase interface shifts the activation loop back to an inactive conformation. Figure 6: The experimental observations of this study are summarized in a graphical model. The Abl KD has a predominantly inactive activation loop conformation that is similar to the conformation once imatinib or other type-2 kinase inhibitors are bound (upper panel). On formation of the SH2–kinase interface, the equilibrium is shifted to a predominantly open activation loop similar to the conformation once dasatinib or other type-1 inhibitors bind to the KD (lower panel). Disruption of the SH2–kinase interface shifts the activation loop back to an inactive conformation. Full size image Using purified Abl SH2–KD unit mutants and conformation-specific Abl kinase inhibitors, we showed that formation of the SH2–kinase interface is a critical switch of activation loop conformation ( Fig. 6 ). Surprisingly, the KD alone, which was previously considered as a reference point for Abl activation, showed profound autophosphorylation impairment with a fully closed activation loop conformation. Initially, this result may appear difficult to reconcile with the high in vitro kinase activity of KD that has been previously observed ( Fig. 1e ) [14] , [26] . In contrast, KD has no effect on total cellular tyrosine phosphorylation in mammalian cells, whereas SH2–KD dramatically increases cellular tyrosine phosphorylation [14] , [17] . These observations support the view that Abl is more reliant on activation loop phosphorylation for its cellular activity when in a competitive cellular environment. Despite the partly deregulated in vitro enzymatic activity, the conformational pre-disposition of a closed activation loop of KD might be detrimental for the normal cellular functions of Abl because of substrate-binding incompatibility. In further support of this model, experiments showed that activation loop phosphorylation is required for the transformation of fibroblasts and hematopoietic progenitors by Bcr–Abl [32] . Therefore, the SH2 domain acts by allosterically enabling autophosphorylation through the induction of an active conformation of the activation loop that is critical for efficient cellular activity. In conjunction with the phosphotyrosine pocket of the SH2 domain, this mechanism also enables the binding and efficient phosphorylation of primed pre-phosphorylated Abl substrates at multiple sites [33] . Importantly, we showed that Abl regulation governed by its SH2 domain can be recapitulated with bacterially expressed proteins in vitro . Our unexpected observation that in vitro Abl autophosphorylation sites strongly overlap with cellular phosphorylation sites does not exclude the possibility of Abl/Bcr–Abl phosphorylation by other tyrosine kinase in cells; however, this finding suggests that autophosphorylation likely plays a pivotal role in the Abl-activation process. These data strengthen the view that Abl converts protein–protein interactions that are mediated via its SH3 or SH2 domains to increase its kinase activity rather than receiving dominant activating signals from upstream tyrosine kinases [9] . An abundant phosphorylation site that we detected was Tyr-245, which replaces the second proline residue in the PxxP motif in the SH2–KD linker of Hck; in addition, Tyr-245 is bound by the SH3 domain and packs into a hydrophobic crevice of the KD [8] . The high level of phosphorylation of Tyr-245 observed in our proteins (all lacking the SH3 domain) suggests a strong phosphorylation consensus and excellent accessibility. While the structural role of Tyr-245 in the inactive conformation is well understood, the consequence of its phosphorylation in the active conformation is unclear. We show that phosphorylation of Tyr-245 is required for full activation loop phosphorylation, suggesting a temporal and functional coupling of Tyr-412 and Tyr-245 phosphorylation. In addition, phosphotyrosine binding by the SH2 domain was required for efficient phosphorylation of Tyr-412, but not of Tyr-245. Efficient activation loop phosphorylation also requires SH2–kinase interactions; thus, it is unlikely that phosphotyrosine-245 will bind to the SH2 domain and stabilize the SH2–kinase interface. While intramolecular binding is sterically possible, a (transient) intermolecular interaction could be envisaged; however, no apparent dimerization of SH2–KD on autophosphorylation was observed ( Supplementary Fig. 1 ). This type of mechanism is difficult to prove without a higher resolution crystal structure of a phosphorylated Abl SH2–KD. Further functional studies are ongoing to provide a reliable mechanistic explanation for these results. The growing arsenal of kinase inhibitors provides valuable chemical tools to better understand kinase signalling. Apart from the elegant work demonstrating allosteric modulation of heterodimeric Raf and EGFR kinases by its inhibitor-bound Braf and Her3 protomers [34] , [35] , we have used type-1 and -2 Abl kinase inhibitors as references to determine the activation loop conformation of the Abl KD in the absence and presence of the SH2 domain. Dasatinib binding converted KD from an inert to an excellent substrate for trans -phosphorylation, which was also observed for specific type-1 inhibitors that target JAK kinases [36] . These results suggest that inhibitor-bound kinases gain some functional properties in cells despite the blockade of their enzymatic activity and that caution is needed when considering the use of activation loop phosphorylation as a reliable marker of kinase activity in the presence of specific kinase inhibitors. We present evidence that mechanisms of Abl activation, which previously relied on time-consuming eukaryotic expression systems, can be mirrored using pure recombinant proteins produced in bacteria. This approach enabled the discovery of a novel mechanism that links the allosteric regulation of the SH2 domain to two critical phosphorylation events and expanded our understanding of Abl kinase activation [37] . Although the ample availability of validated research tools, such as antibodies, kinase inhibitors and mutations, has accelerated this process, the proposed workflow and experimental approaches will facilitate future quantitative analyses of allosteric regulatory mechanisms in other tyrosine kinases. Protein expression and purification Numbering for the spliceform 1b of the human ABL1 gene is used throughout the manuscript. Complementary DNAs encoding for the human Abl protein (Abl KD (KD): residues 248–534, Abl SH2–KD unit (SH2–KD): residues 138–534) were cloned into the NheI (5′) and XhoI (3′) restriction sites of pET-21d (Merck Millipore) containing a carboxy-terminal hexa-histidine affinity tag with the following primers: AblSH2_sense_NheI: 5′- CGGGCTAGCGTCAACAGTCTGGAGAAACAC -3′, AblKD_sense_NheI: 5′- CGGGCTAGCTCCCCCAACTACGACAAGTGG -3′ and Abl(SH2–)KD_antisense_XhoI: 5′- GCGCTCGAGGACGCCTTGTTTCCCCAGCTC -3′. For the experiments shown in Fig. 5d , a 2xMyc-SBP tag (amino-acid sequence: LEEQKLISEEDLGSEQKLISEEDLGS DEKTTGWRGGHVVEGLAGELEQLRARLEHHPQGQREPGSVD) was cloned into the XhoI and SalI site of pET-21d using a synthetic gene cassette (custom gene synthesis by GenScript), thereby adding the additional tag to the C terminus of the Abl SH2–KD protein. The Quickchange site-directed mutagenesis kit (Stratagene) and complementary oligonucleotides (only sense oligonucleotide sequence is shown, changed nucleotides are underlined) were used to introduce point mutations (I164E: 5′- CTGAGCAGCGGGGAGAATGGCAGCTTC -3′, T231R: 5′- GCTCATCACCAGGCTCCATTATCC -3′, S173N: 5′- GGTGCGTGAGAATGAGAGCAGTC -3′, Y412F: 5′- GGGGACACCTTCACAGCCCATGC -3′, Y245F: 5′- CAAGCCCACTGTCTTCGGTGTGTCCC -3′ and D382N: 5′- CTTCATCCACAGAAACCTTGCTGCCCGAAACTG -3′) and combinations of these mutations. Abl KD and SH2–KD proteins were co-expressed with the YopH phosphatase in E. coli BL21(DE3) by co-transformation of pCDFDuet-1-YopH and pET-21d-Abl KD or SH2–KD plasmids. Liquid cultures in Terrific Broth (TB) medium supplemented with carbenicillin and streptomycin (50 μg ml −1 each) were grown to an OD 600 nm of 1.2. Protein expression was induced by addition of isopropyl-b- D -thiogalactoside for 10–16 h at 18 °C. Cells were harvested by centrifugation, resuspended in 50 mM Tris-HCl, pH 7.5/500 mM NaCl/20 mM imidazole/5% glycerol/1 mM dithiothreitol (DTT) and lysed by three cycles of homogenization at 15,000 p.s.i. in Avestin Emulsiflex. Protein purification was carried out using the C-terminal hexa-histidine tag by nickel-affinity chromatography (5 ml His-Trap column). Bound proteins were eluted with a gradient from 20 to 500 mM imidazole over five column volumes. Protein was further purified to remove YopH phosphatase and other contaminants by anion-exchange chromatography on a 1 ml MonoQ 5/50 GL, and eluted with a linear gradient of 0–35% buffer B (20 mM Tris-HCl, pH7.5/1 M NaCl/5% glycerol/1 mM DTT). Final samples were dialyzed against 20 mM Tris-HCl, pH 7.5/150 mM NaCl/5% glycerol/1 mM DTT. Protein identity was confirmed by mass spectrometry. Multi-angle light scattering Multi-angle light scattering was used to probe for protein quality and oligomerization states. All measurements were performed at room temperature using a DAWN HELLIOS Multi-angle light-scattering detector (Wyatt Technology, Santa Barbara, CA) online with a size-exclusion chromatography column. Eighty μl at a concentration of 0.5 mg ml −1 of purified recombinant proteins was injected onto a Superdex 75 HR10/30 column (GE Healthcare) in size exclusion chromatography (SEC) buffer (25 mM Tris-HCl, pH 7.5/100 mM NaCl/5% glycerol/1 mM DTT) and eluted at a flow rate of 0.5 ml min −1 . Absolute molecular weights and homogeneity were determined using ASTRA version 5.3 from Wyatt Technologies. In vitro kinase assays One ng of recombinant KD or SH2–KD protein, 75 μM ATP, 7 μCi γ- 32 P-ATP was incubated with a peptide with an optimal Abl substrate sequence carrying an N-terminal biotin (biotin-GGEAIYAAPFKK-amide) in kinase assay buffer (20 mM Tris-HCl, pH 7.5/5 mM MgCl 2 /1 mM DTT/10 μM bovine serum albumin) for 12 min at room temperature in a final assay volume of 20 μl. Peptide concentrations ranged from 3.125 to 100 μM. The terminated reaction (10 μl 7.5 M guanidine hydrochloride) was spotted onto a SAM2 Biotin Capture membrane (Promega) and further treated according to the instructions of the manufacturer by washing four times with 2 M NaCl, followed by four times with 2 M NaCl/1% H 3 PO 4 , two times in distilled water and finally shortly rinsed with ethanol before drying the membranes and quantification of incorporated radioactivity in a liquid scintillation counter. Small-angle X-ray scattering Synchrotron SAXS data were collected at EMBL P12 beamline (DESY, Hamburg) [38] , [39] and recorded at 10 °C using a PILATUS 1M pixel detector (DECTRIS) at a sample–detector distance of 2.7 m and a wavelength of ~1.2 Å. This set-up covers a range of momentum transfer of 0.005< s <0.6 Å −1 ( s =4 π sin( θ ) λ −1 , where 2 θ is the scattering angle). A robotic sample changer [40] was used and the samples were measured in a concentration range from 4.52 to 0.66 mg ml −1 (4.52, 2.66, 1.33 and 0.66 mg ml −1 ) for KD and SH2–KD wt and from 1.3 to 0.37 mg ml −1 (1.3, 0.75 and 0.35 mg ml −1 ) for SH2–KD I164E. Initial data pre-processing and reduction were performed using an automatic pipeline and theoretical extrapolation to infinite dilution made for the analysis. For the calculation of the forward scattering I (0) and the radius of gyration ( R g ), the Guinier approximation implemented in PRIMUS [41] was used, assuming that at very small angles ( s <1.3/ R g ) the intensity is represented as I ( s )= I (0) exp(−( sR g ) 2 3 −1 ). The pair-distance distribution function P ( r ) was evaluated with GNOM [42] , and consecutively the maximum particle dimension ( D max ) as well as R g were estimated. Moreover, the Porod volume was computed using the Porod invariant [43] , and the molecular mass estimated [44] . Ab initio models were computed with DAMMIF [45] , using low-resolution data in the range of 0.012< s <0.20 Å −1 . The algorithm constructs bead models yielding a scattering profile with the lowest possible discrepancy ( χ ) to the experimental data while keeping beads interconnected and the model compact. Twenty independent ab initio reconstructions were performed and then averaged using DAMAVER [46] , which also provides a value of normalized spatial discrepancy, representing a measure of similarity among different models. Model superimposition was computed using the program SUPCOMB [47] . Rigid body modelling was performed using the software BUNCH. Flexibility was assessed with the software Ensemble Optimization Method 2.0 (ref. 48 )—an enhanced version of Ensemble Optimization Method (EOM) [49] —which assumes coexistence of a range of conformations in solution for which an average scattering intensity fits the experimental SAXS data. Using EOM 2.0, a pool of 10,000 independent models is initially generated. The theoretical scattering curve is automatically computed for each model in the pool by using CRYSOL [50] . Afterwards, a genetic algorithm is employed to selected ensembles, randomly distributed in terms of size from 5 to 20 conformers, by calculating the average theoretical profiles and fitting them to the experimental SAXS data. The genetic algorithm is hence repeated 100 times, and the ensemble with the lowest discrepancy is reported as the best solution out of 100 final ensembles. Autophosphorylation assays Autophosphorylation assays were carried out with 265 nM of recombinant Abl proteins in 20 mM Tris-HCl, pH 7.5/5 mM MgCl 2 /1 mM DTT/300 μM ATP in a total volume of 50 μl. Reactions were stopped at desired time points by adding 50 μl of 2 × SDS–PAGE sample buffer. Thirty percent of the total reaction volume was dot blotted on a nitrocellulose membrane using the BioDot Apparatus (Bio-Rad) system following the manufacturers’ recommendations. Total phosphotyrosine (clone 4G10, Millipore, diluted 1:2,000 in Odyssey blocking buffer-PBS (Li-cor Biosciences)), pY245 (2868S, Cell Signaling, diluted 1:1,000 in Odyssey blocking buffer-PBS (Li-cor Biosciences)) or pY412 (2865S, Cell Signaling, diluted 1:1,000 in Odyssey blocking buffer-PBS (Li-cor Biosciences)) levels were quantified using the Li-cor Odyssey imaging system and normalized for total Abl protein levels (Penta-His antibody, Qiagen, diluted 1:3,000 in Odyssey blocking buffer-PBS (Li-cor Biosciences)) co-incubated with the phosphotyrosine antibodies. Abl proteins incubated without ATP were used as background and subtracted before normalizing values by dividing phosphorylation signal by penta-His signal. Normalized values were plotted over incubation time and initial slopes of linear fits were calculated. The slope of SH2–KD wt was set to 1.0 to compare autophosphorylation velocities of different SH2–KD mutants from independent experiments. Trans -autophophorylation assays Pairs of active and catalytically deficient KD and SH2–KD protein were mixed in a 1:1 molar ratio at 265 nM final concentration in 50 μl volume in 20 mM Tris-HCl, pH 7.5/5 mM MgCl 2 /1 mM DTT/300 μM ATP. Reactions were stopped at desired time points by adding 50 μl of 2 × SDS–PAGE sample buffer. Thirty percent of the total reaction volume was resolved on 12% SDS–PAGE gels, transferred onto a nitrocellulose membrane by semidry electroblotting and incubated with total phosphotyrosine (4G10, Millipore), pY245 (2868S, Cell Signalling) or pY412 (2865S, Cell Signalling) antibodies mixed with a Penta-his antibody (Qiagen) under the same conditions as described above for the autophosphorylation assays. Quantification using the Li-cor Odyssey imaging system and data analysis were also performed using the same workflow as described above Abl–drug complexes Abl KD and SH2–KD complexes with imatinib and dasatinib were obtained by incubating the recombinant proteins with a three-fold molar excess of imatinib or dasatinib (Symansis; stock solutions of 10 mM in dimethylsulphoxide) for 10 min at room temperature, followed by extensive dialysis against 20 mM Tris-HCl, pH 7.5/150 mM NaCl/5% glycerol/1 mM DTT to remove free drug. The final dialyzed proteins were used as substrate for the trans -phophorylation assays in Fig. 5 . How to cite this article: Lamontanara, A. J. et al . The SH2 domain of Abl kinases regulates kinase autophosphorylation by controlling activation loop accessibility. Nat. Commun. 5:5470 doi: 10.1038/ncomms6470 (2014).